Microbiota and host determinants of behavioural phenotype in maternally separated mice Early-life stress is a determinant of vulnerability to a variety of disorders that include dysfunction of the brain and gut. Here we exploit a model of early-life stress, maternal separation (MS) in mice, to investigate the role of the intestinal microbiota in the development of impaired gut function and altered behaviour later in life. Using germ-free and specific pathogen-free mice, we demonstrate that MS alters the hypothalamic–pituitary–adrenal axis and colonic cholinergic neural regulation in a microbiota-independent fashion. However, microbiota is required for the induction of anxiety-like behaviour and behavioural despair. Colonization of adult germ-free MS and control mice with the same microbiota produces distinct microbial profiles, which are associated with altered behaviour in MS, but not in control mice. These results indicate that MS-induced changes in host physiology lead to intestinal dysbiosis, which is a critical determinant of the abnormal behaviour that characterizes this model of early-life stress. Traumatic events in childhood have been associated with the development of psychiatric diseases [1] and functional bowel disorders [2] later in life. Maternal separation (MS) in rodents is a well-established model of early-life stress that induces long-lasting alterations in behaviour [3] , [4] and gut dysfunction [5] , mimicking many features of irritable bowel syndrome [6] . MS induces hyper-responsiveness of the hypothalamic–pituitary–adrenal (HPA) axis [7] , depression and anxiety-like behaviour [8] , [9] , increased vulnerability of cholinergic neurons to immunotoxic insult [10] , visceral hypersensitivity [11] , [12] , [13] and increased intestinal permeability [14] , [15] , [16] , [17] in adulthood. Furthermore, MS pups have altered cholinergic activity with increased expression of choline acetyltransferase in the gut [15] . MS is also associated with abnormal gut microbiota composition [18] , and probiotics seem to ameliorate changes in gut and brain induced by early-life stress [19] , [20] , [21] . There is growing evidence that intestinal microbiota can affect host behaviour [22] . The absence of bacteria results in an abnormal HPA response to stress that can be reversed by colonization with commensal bacteria [23] . Germ-free (GF) mice display higher exploratory and lower anxiety-like behaviours, as well as altered levels of neurotrophins and multiple genes involved in synaptic long-term potentiation and second messenger pathways [24] , [25] . Microbial colonization during early-life also regulates the hippocampal serotonergic system [26] . Furthermore, perturbing gut microbiota in conventional mice results in increased exploratory behaviour and differential expression of brain-derived neurotrophic factor (BDNF) in the amygdala and hippocampus [27] . However, no study has explored the role of the intestinal microbiota in the altered behavioural phenotype that is a consequence of early-life stress. Therefore, the aim of this study was to investigate the relative contributions of gut commensal bacteria as well as host factors in the expression of altered behaviour in the MS model. Here we show that MS induces changes in host physiology that alter colonic milieu and lead to intestinal dysbiosis, which then triggers, likely through production of microbial metabolites, the abnormal behaviour that characterizes this model of early-life stress. Corticosterone and colonic acetylcholine release Analysis of data from specific pathogen-free (SPF) and all (male and female) GF mice with a two-way analysis of variance (ANOVA), with one factor being the presence/absence of gut microbiota (SPF versus GF) and the second factor being the treatment (MS versus control), showed a significant effect of MS ( F (1,35)=22.33, P <0.001) for serum corticosterone levels ( Fig. 1a ), colonic acetylcholine (Ach) release after KCl ( F (1,79)=5.60, P =0.020) ( Fig. 1b ), and electrical field stimulation (EFS) ( F (1,77)=16.32, P <0.001; Fig. 1c ), and a significant effect of the presence/absence of microbiota for KCl stimulation ( F (1,79)=63.52, P <0.001). 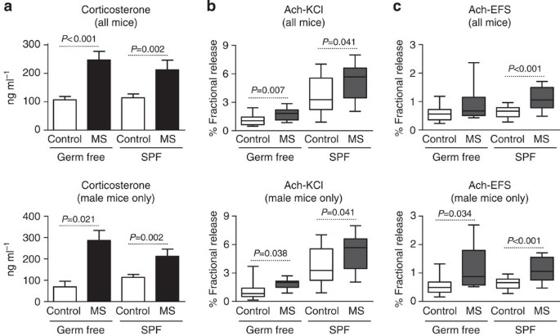Figure 1: MS leads to elevated corticosterone and colonic acetylcholine release in SPF and GF mice. (a) Serum corticosterone levels in all SPF and GF MS and control mice (SPF MS,n=13; SPF control,n=20; GF MS,n=13; GF control,n=16, upper panel), and male only SPF and GF MS and control mice (SPF MS,n=13; SPF control,n=20; GF MS,n=7; GF control,n=6, lower panel). The graphs represent mean±s.e.m. (b,c) Acetylcholine release from colon tissues induced by KCl or EFS administration in SPF (right) and GF (left) MS and control mice (SPF MS,n=13; SPF control,n=20; GF MS,n=13; GF control,n=16), and male only SPF and GF MS and control mice (SPF MS,n=13; SPF control,n=20; GF MS,n=7; GF control,n=6, lower panel). The graphs represent median (IQD). The assessment of the main effects (presence/absence of gut microbiota and MS) was performed with two-way ANOVA. If a statistically significant effect of one of the categorical variables was observed, at-test within groups was performed. Figure 1: MS leads to elevated corticosterone and colonic acetylcholine release in SPF and GF mice. ( a ) Serum corticosterone levels in all SPF and GF MS and control mice (SPF MS, n =13; SPF control, n =20; GF MS, n =13; GF control, n =16, upper panel), and male only SPF and GF MS and control mice (SPF MS, n =13; SPF control, n =20; GF MS, n =7; GF control, n =6, lower panel). The graphs represent mean±s.e.m. ( b , c ) Acetylcholine release from colon tissues induced by KCl or EFS administration in SPF (right) and GF (left) MS and control mice (SPF MS, n =13; SPF control, n =20; GF MS, n =13; GF control, n =16), and male only SPF and GF MS and control mice (SPF MS, n =13; SPF control, n =20; GF MS, n =7; GF control, n =6, lower panel). The graphs represent median (IQD). The assessment of the main effects (presence/absence of gut microbiota and MS) was performed with two-way ANOVA. If a statistically significant effect of one of the categorical variables was observed, a t -test within groups was performed. Full size image In SPF MS mice, serum corticosterone levels were 1.9-fold higher compared with SPF controls ( Fig.1a ). Superfusion experiments demonstrated that colonic Ach release was increased 1.9- and 1.5-fold in SPF MS mice compared with SPF controls after neuronal EFS and KCl stimulation, respectively ( Fig. 1b,c ). While EFS is indicative of neuronal function, KCl stimulation assesses total amount of stored Ach. In all GF mice, serum corticosterone levels were 2.3-fold higher in MS mice compared with GF controls ( Fig. 1a ). These differences were not gender dependent as two-way ANOVA showed significant effect of MS ( F (1,21)=20.263, P <0.001) but not of gender. When analysing only GF male mice (controls and MS), we observed a significant effect of MS on serum corticosterone levels ( F (1,8)=8.10, P =0.022) ( Fig. 1a , lower panel). In all GF mice, MS induced higher colonic KCl-stimulated acetylcholine release compared with controls ( Fig. 1b ) and a similar trend was observed after EFS ( Fig. 1c ). When analysing only GF male mice (controls and MS), we confirmed a significant effect of MS on colonic Ach release by KCl ( Fig. 1b , lower panel), and observed a statistical difference in EFS ( F (1,18)=5.24, P =0.034) ( Fig. 1c , lower panel). Overall, GF mice released less Ach in response to KCl stimulation than SPF mice ( Fig. 1b ). MS altered the colonic microbiota composition of SPF mice We used a 16S ribosomal DNA-based method, denaturing gradient gel electrophoresis (DGGE), to screen colonic microbiota composition profiles. MS was associated with an altered microbiota profile in 4-week-old MS mice, compared with controls ( Supplementary Fig. 1b ). These differences in microbiota composition were maintained in adult mice at 20 weeks of age ( Supplementary Fig. 1a ). Using Dice coefficient and UPGMA (unweighted pair group method with arithmetic mean) group method, MS mice samples clustered separately from control mice samples, sharing only 55–70% similarity. These results were confirmed by partial 16S rRNA gene profiling using Illumina sequencing, as shown in Fig. 2 . The relative abundance of operational taxonomic units (OTUs) is plotted in an ordination-organized heat map ( Fig. 2a , left) and a principal coordinate plot of the Morisita–Horn dissimilarity matrix based on proportional abundance of OTUs in each sample ( Fig. 2a , right). Several OTUs were increased in abundance in MS mice (OTU nos. 143, 597,506,173 and 762). The complete list of OTUs and respective sequences that differed between control and MS mice is shown in Supplementary Table 1 . Analysis of the taxonomic composition at the highest assigned taxonomic level ( Supplementary Fig. 2a , at phylum level; Supplementary Fig. 3 , at genus level) showed that MS mice presented with higher abundance of unclassified Lachnospiraceae and lower abundance of the genus Mucispirillum (Deferribacteraceae) (all corrected P <0.0001; Fig. 2b ). These results indicate that MS induces early-life dysbiosis, which persists into adulthood. 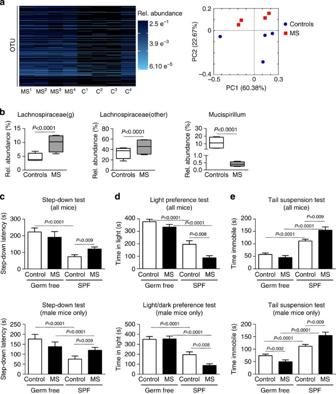Figure 2: MS induced colonic dysbiosis and anxiety-like behaviour in SPF but not in GF mice. (a) OTUs distribution at phylum level plotted in an ordination-organized heat map (based on Bray Curtis distance metric) of SPF MS and control mice (left panel). The data are normalized to proportional abundances and are represented by the intensity (blue) for each OTU. On the right, PCoA ordination plot of Morisita–Horn dissimilarity matrix calculated with QIIME on direct read counts of SPF MS and control mice. (b) Taxonomic composition of SPF MS and control mice colonic microbiota: main genera contributing to the taxonomic differences between SPF MS and control mice. ThePvalues obtained from the comparison between groups (controls versus MS) were corrected with the ‘FDR’ method, accepting a 3% FDR. (c) Latency to step down from an elevated platform, total time spent in the illuminated compartment (d), and total duration of immobility during tail suspension test (e) in SPF (right) and GF (left) MS and control mice (upper panel; SPF MS,n=13; SPF control,n=20; GF MS,n=37 (25 males and 12 females); GF control,n=54 (26 males and 28 females) for step-down and light preference tests; SPF MS,n=13; SPF control,n=20; GF MS,n=23 (15 males and 8 females); GF control,n=35 (15 males and 20 females) for tail suspension test), and in male mice only (lower panel). The graphs represent mean±s.e.m. The assessment of the main effects (presence/absence of gut microbiota and MS) was performed with two-way ANOVA. If a statistically significant effect of one of the categorical variables was observed, at-test within groups was performed. Rel., relative. Figure 2: MS induced colonic dysbiosis and anxiety-like behaviour in SPF but not in GF mice. ( a ) OTUs distribution at phylum level plotted in an ordination-organized heat map (based on Bray Curtis distance metric) of SPF MS and control mice (left panel). The data are normalized to proportional abundances and are represented by the intensity (blue) for each OTU. On the right, PCoA ordination plot of Morisita–Horn dissimilarity matrix calculated with QIIME on direct read counts of SPF MS and control mice. ( b ) Taxonomic composition of SPF MS and control mice colonic microbiota: main genera contributing to the taxonomic differences between SPF MS and control mice. The P values obtained from the comparison between groups (controls versus MS) were corrected with the ‘FDR’ method, accepting a 3% FDR. ( c ) Latency to step down from an elevated platform, total time spent in the illuminated compartment ( d ), and total duration of immobility during tail suspension test ( e ) in SPF (right) and GF (left) MS and control mice (upper panel; SPF MS, n =13; SPF control, n =20; GF MS, n =37 (25 males and 12 females); GF control, n =54 (26 males and 28 females) for step-down and light preference tests; SPF MS, n =13; SPF control, n =20; GF MS, n =23 (15 males and 8 females); GF control, n =35 (15 males and 20 females) for tail suspension test), and in male mice only (lower panel). The graphs represent mean±s.e.m. The assessment of the main effects (presence/absence of gut microbiota and MS) was performed with two-way ANOVA. If a statistically significant effect of one of the categorical variables was observed, a t -test within groups was performed. Rel., relative. Full size image MS induced anxiety-like behaviour in SPF but not in GF mice Mouse behaviour was assessed using step-down, light preference and tail suspension tests ( Fig. 2c–e ). When analysed with two-way ANOVA, we observed a significant effect of the presence/absence of gut microbiota for all three behavioural tests, step-down ( F (1,182)=13.06, P <0.001), tail suspension ( F (1,77)=79.85, P <0.001) and light preference ( F (1,123)=57.10, P <0.001) tests. We also found a significant interaction between MS and presence/absence of microbiota for step-down ( F (1,182)=4.04, P =0.046) and tail suspension ( F (1,77)=8.90, P =0.004) tests, and a significant effect of MS for the light preference test ( F (1,123)=7.127, P =0.009). When analysing only male mice, we observed a significant effect of the presence/absence of gut microbiota for all three behavioural tests, the step-down ( F (1,92)=8.4, P =0.005), tail suspension ( F (1,49)=67.56, P <0.001) and light preference ( F (1,83)=47.96, P <0.001) tests. We also found a significant interaction between MS and presence/absence of microbiota for the step-down ( F (1,92)=4.06, P =0.047) and tail suspension ( F (1,49)=15, P <0.001) tests. When analysing GF and SPF mice separately, we found that MS induced anxiety-like behaviour in SPF mice as MS mice stepped down from the elevated platform with latency delayed by 70% compared with controls ( Fig. 2c ). Likewise, SPF MS mice spent 55% less time in the illuminated compartment ( Fig. 2d ) and displayed longer latency to re-enter the illuminated compartment compared with controls ( P <0.03). Finally, in the tail suspension test, SPF MS mice were immobile for a longer time compared with control mice ( P =0.0091; Fig. 2e ). In contrast, MS did not induce anxiety-like behaviour in GF mice; responses in the step-down, light preference and tail suspension tests were similar in MS and control GF mice ( Fig. 2c–e ). To further characterize the effect of MS on exploratory and locomotor behaviour in GF conditions, we performed the open-field test. MS GF mice spent similar amount of time in the centre of the arena and travelled similar distance as the controls ( Supplementary Fig. 4 ). However, the number of faecal pellets excreted by GF MS mice (4.75±0.96) during the open-field test was greater than that of controls (2.47±1.58, P =0.012) indicative of enhanced stress-induced colonic motility [28] , [29] . No gender effect or its interaction with MS was found when testing the data from GF mice with a two-way ANOVA. In GF male mice only (controls and MS), we confirmed no effect of MS on the light preference, open-field and step-down tests, but increased faecal output in MS mice during the open-field test ( F (1,20)=16.36, P =0.001). Interestingly, we observed a significant effect of MS on the tail suspension test ( F (1,28)=5.86, P =0.022), although in the opposite direction than in SPF MS mice ( Fig. 2e ), as GF MS male mice ( n =15) spent less time immobile than controls ( n =15), suggesting that MS in GF conditions confers some protection from behavioural despair. It is well established that GF mice behave differently than conventional mice [24] , [25] , [26] , [27] . In our experiments, control GF mice took longer to step down from the elevated platform when compared with control SPF mice and they spent longer time in the illuminated area ( Fig. 2c,d ). Brain BDNF and catecholamine levels Two-way ANOVA analysis showed a significant effect of MS ( F (1,33)=10.73, P =0.002) on hippocampal BDNF levels, while the presence of gut microbiota had a significant effect on hippocampal serotonin ( F (1,13)=7.61, P =0.016), BDNF ( F (1,33)=19.61, P <0.001) and noradrenaline ( F (1,14)=235.240, P <0.001) levels. We also observed a significant interaction between MS and presence of gut microbiota on hippocampal BDNF levels ( F (1,33)=7.51, P =0.010): this interaction was mainly driven by the effect of MS in GF mice. When analysing the two groups separately, SPF MS and control mice had similar levels of BDNF, serotonin, dopamine and noradrenaline ( Fig. 3a–e ). However, GF MS mice exhibited higher hippocampal BDNF levels than GF controls. When analysing these BDNF data with a two-way ANOVA, we did not observe any significant effect of gender ( F (1,12)=0.020, P =0.891) or its interaction with MS. Similarly, we found no significant effect of gender, MS, or their interaction on any of the other neurotransmitters measured. When analysing only GF male mice (controls and MS), we confirmed a significant effect of MS on hippocampal BDNF levels ( F (1,9)=20.98, P =0.001) and no effect of MS on other neurotransmitters. 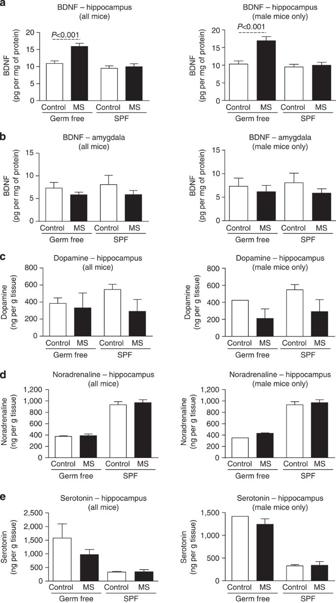Figure 3: MS alters levels of hippocampal BDNF in GF mice only. Total free BDNF levels in brain sections of hippocampus (a) and amygdala (b) of GF (left) and SPF (right) mice (SPF MS,n=5; SPF control,n=5; GF MS,n=5 (2 males and 3 females); GF control,n=5 (3 males and 2 females)). Dopamine (c) noradrenaline (d), and serotonin (e) levels in brain sections of hippocampus of GF (left) and SPF (right) mice (SPF MS,n=5; SPF control,n=5; GF MS,n=5 (3 males and 2 females); GF control,n=5 (2 males and 3 females)). The graphs represent mean±s.e.m. The assessment of the main effects (presence/absence of gut microbiota and MS) was performed with two-way ANOVA. If a statistically significant effect of one of the categorical variables was observed, at-test within groups was performed. Figure 3: MS alters levels of hippocampal BDNF in GF mice only. Total free BDNF levels in brain sections of hippocampus ( a ) and amygdala ( b ) of GF (left) and SPF (right) mice (SPF MS, n =5; SPF control, n =5; GF MS, n =5 (2 males and 3 females); GF control, n =5 (3 males and 2 females)). Dopamine ( c ) noradrenaline ( d ), and serotonin ( e ) levels in brain sections of hippocampus of GF (left) and SPF (right) mice (SPF MS, n =5; SPF control, n =5; GF MS, n =5 (3 males and 2 females); GF control, n =5 (2 males and 3 females)). The graphs represent mean±s.e.m. The assessment of the main effects (presence/absence of gut microbiota and MS) was performed with two-way ANOVA. If a statistically significant effect of one of the categorical variables was observed, a t -test within groups was performed. Full size image No overt gut inflammation in MS mice Body weight was similar between MS and controls in SPF conditions. No overt inflammation was found in SPF mice as there was no difference in myeloperoxidase (MPO) activity assay or acute and chronic inflammatory infiltrates in the colon of MS and control mice. Similarly, body weight was similar between MS and controls in GF conditions. No overt inflammation was found in GF MS or control mice, as reflected by similar MPO activity in these groups (0.98±1.53 versus 0.4±0.28 per mg of tissue) and by the absence of an acute or chronic inflammatory infiltrate in the colon. Similarly, no differences were detected in serum C-reactive protein (CRP) levels between GF MS (4.58±1.33 ng ml −1 ) and GF controls (5.31±1.83 ng ml −1 ). Colonization of adult GF MS and control mice We next examined the impact of microbial colonization of GF MS and control mice using microbiota from an SPF mouse that had not been subjected to MS (SPF control mouse). Colonization of both control and MS mice was performed by short-term cohabitation with a single SPF control mouse (two SPF control mice were used for two rounds of colonization experiments). 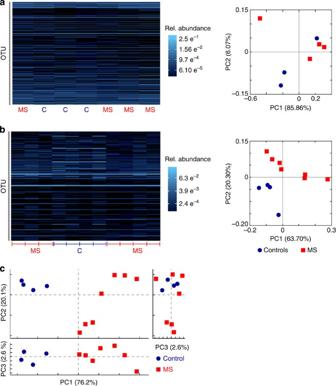Figure 4: Colonization of adult GF mice results in different colonic microbial profiles in MS and control mice. OTUs distribution at phylum level plotted in an ordination-organized heat map (based on Bray Curtis distance metric) of GF MS and control mice colonized by cohabitation with a single SPF donor: Donor 1 (a) and donor 2 (b) (left panels). The data are normalized to proportional abundances and are represented by the intensity (blue) for each OTU. On the right, PCoA ordination plot of Morisita–Horn dissimilarity matrix calculated with QIIME on direct read counts of GF MS and control mice that were colonized by cohabitation with a single SPF donor: Donor 1 (a) and donor 2 (b) (right panels). (c) PICRUSt prediction of metagenomic functional content of 16S rRNA of germ-free MS and control mice colonized by cohabitation with a single SPF donor. Figure 4a,b illustrates OTUs distribution at phylum level of colonized MS and control mice (donor 1, Fig. 4a ; donor 2, Fig. 4b ), plotted in an ordination-organized heat map and principal coordinates analysis (PCoA) ordination of the samples calculated from the Morisita–Horn dissimilarity metric. permutational multivariate analysis of variance (PERMANOVA) analysis of the distance matrix calculated with Bray Curtis method on normalized data (all samples were subsampled to the same depth) with the script compare_categories.py showed a statistically significant difference between colonized MS and control mice ( P =0.002) that was reflected in the ordinated heat maps and in the ordination plots. Similar results were observed when analysing the Morisita–Horn dissimilarity matrix ( P =0.03). The analysis of the taxonomic composition ( Supplementary Fig. 2b , summary at phylum level) showed that several OTUs were increased in control mice, including those pertaining to the family Lachnospiraceae (OTU nos. 4, 6, 7, 21, 56 and 63; corrected P <0.0001–0.043), one from the genus Clostridium (Lachnospiraceae, OTU no. 10; corrected P =0.049) and one belonging to the genus Atopobium (OTU no. 122; corrected P =0.02). The complete list of OTUs and how their sequences are different between MS and control mice is shown in Supplementary Table 2 . Figure 4: Colonization of adult GF mice results in different colonic microbial profiles in MS and control mice. OTUs distribution at phylum level plotted in an ordination-organized heat map (based on Bray Curtis distance metric) of GF MS and control mice colonized by cohabitation with a single SPF donor: Donor 1 ( a ) and donor 2 ( b ) (left panels). The data are normalized to proportional abundances and are represented by the intensity (blue) for each OTU. On the right, PCoA ordination plot of Morisita–Horn dissimilarity matrix calculated with QIIME on direct read counts of GF MS and control mice that were colonized by cohabitation with a single SPF donor: Donor 1 ( a ) and donor 2 ( b ) (right panels). ( c ) PICRUSt prediction of metagenomic functional content of 16S rRNA of germ-free MS and control mice colonized by cohabitation with a single SPF donor. Full size image We then analysed the composition at the highest assigned taxonomic level and found that MS mice had lower abundance of unclassified Lachnospiraceae (corrected P <0.0001) and higher abundance of the genus Blautia (Lachnospiraceae; corrected P <0.0001), the genus Parabacteroides (corrected P <0.0001) and Lactobacillus ( P <0.0001; Supplementary Fig. 5a,b ). This demonstrates that the microbial composition of MS mice and control mice at 3 weeks post colonization differed despite being colonized with the same donor, in agreement with the initial DGGE screen ( Supplementary Fig. 1c ). To assess whether these differences in microbiota profiles could have any significant impact on their metabolic activity, we used PICRUSt [30] . Interestingly, inferred metagenomic profiles were strikingly different between colonized MS and control mice ( Fig. 4c ). We found differences in multiple specific metabolic pathways, including the metabolism of glutamate and glutamatergic synapse, phenylalanine, tryptophan, tyrosine and fatty acids ( Supplementary Data 1 ). These molecules have a direct link to the central nervous system (CNS), and thus could explain the behavioural differences between colonized control and MS mice. Colonization altered the behaviour of MS mice only Bacterial colonization of GF mice induced anxiety-like behaviour and behavioural despair in MS mice but not in controls ( Fig. 5 ), as assessed by step-down and tail suspension tests at 3 weeks post colonization. The data were analysed with mixed two-way repeated measures ANOVA, where the between-subjects categorical variable was ‘treatment’ (MS or control) and the within-subjects categorical variable was ‘colonization’ (before and after colonization) and gender. A significant interaction between colonization and MS was observed for the step-down ( F (1,18)=6.25, P =0.022) and tail suspension tests ( F (1,18)=9.161, P =0.007) but not for the light preference test ( F (1,18)=0.160, P =0.694). MS mice displayed longer latency to step down from the elevated platform compared with before colonization, whereas control mice did not alter their behaviour ( Fig. 5a ). Similarly, colonized MS mice, but not controls, spent more time immobile during the tail suspension test compared with before colonization ( Fig. 5b ). A significant effect of colonization alone was observed for the light preference test ( F (1,18)=40.61, P <0.001) as the time spent in the light decreased after colonization in both controls and MS mice ( Fig. 5c ). When examining the behaviour of individual mice before and after the colonization (delta values, Supplementary Fig. 6 ), we observed a statistically significant difference between MS and control mice for both step-down ( P =0.035) and tail suspension tests ( P =0.002), but not for the light preference test. No behavioural differences were detected between control and MS mice using the open-field test. 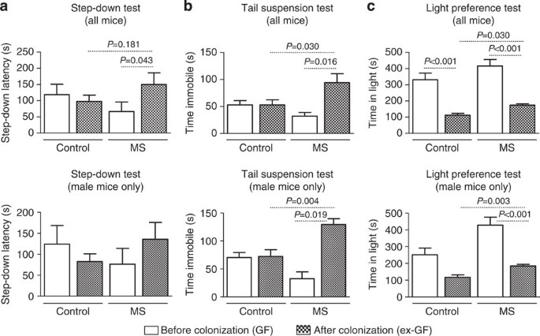Figure 5: Colonization of adult GF mice induces anxiety-like behaviour and behavioural despair in MS mice but not in controls. Latency to step down from an elevated platform in control and MS mice (upper panel), and in male mice only (lower panel), before (GF) and after colonization (ex-GF) by cohabitation with a single SPF donor. (a) Total duration of immobility during the tail suspension test in GF and colonized control and MS mice (upper panel), and in male mice only (lower panel). (b) Total time spent in the illuminated compartment during the light preference test in GF and colonized control and MS mice (upper panel), and in male mice only (lower panel). (c) MS,n=11, 7 males and 4 females; control,n=16, 9 males and 7 females. The graphs represent mean±s.e.m. The data were analysed with mixed two-way repeated measures ANOVA, where the between-subjects categorical variable was ‘treatment’ (MS or control) and the within-subjects categorical variable was ‘colonization’ (before or after colonization). If a statistically significant effect of one of the categorical variables was observed, at-test within groups was performed. Figure 5: Colonization of adult GF mice induces anxiety-like behaviour and behavioural despair in MS mice but not in controls. Latency to step down from an elevated platform in control and MS mice (upper panel), and in male mice only (lower panel), before (GF) and after colonization (ex-GF) by cohabitation with a single SPF donor. ( a ) Total duration of immobility during the tail suspension test in GF and colonized control and MS mice (upper panel), and in male mice only (lower panel). ( b ) Total time spent in the illuminated compartment during the light preference test in GF and colonized control and MS mice (upper panel), and in male mice only (lower panel). ( c ) MS, n =11, 7 males and 4 females; control, n =16, 9 males and 7 females. The graphs represent mean±s.e.m. The data were analysed with mixed two-way repeated measures ANOVA, where the between-subjects categorical variable was ‘treatment’ (MS or control) and the within-subjects categorical variable was ‘colonization’ (before or after colonization). If a statistically significant effect of one of the categorical variables was observed, a t -test within groups was performed. Full size image When analysing the effect of gender, we found a statistically significant interaction between bacterial colonization and gender for the tail suspension test ( F (1,18)=23.85, P <0.001) but not for step-down or light preference tests ( Fig. 5 ). Analysing only GF male mice (controls and MS), we confirmed a significant interaction between colonization and MS for the tail suspension test ( Fig. 5 ). When examining the behaviour of individual male mice before and after colonization (delta values, Supplementary Fig. 6 ), we observed a statistically significant difference between MS and control male mice for both step-down ( P =0.018) and tail suspension tests ( P <0.001), and a similar trend for the light preference test ( P =0.086). No behavioural differences were detected between control and MS mice using the open-field test. There was no statistically significant effect of MS on BDNF, noradrenaline or serotonin levels in the hippocampus and amygdala of colonized mice ( Supplementary Fig. 7a–h ); however, MS affected dopamine levels in the hippocampus ( F (1,3)=27.2, P =0.014) and amygdala ( F (1,3)=25.77, P =0.015). When analysing only male mice, we did not observe any effect of MS on any of the studied neurotransmitters. Microbiota transfer into control GF mice To determine whether the altered microbiota associated with MS mice is sufficient to induce the MS behavioural phenotype, we colonized adult control GF mice with microbiota from SPF MS or control mice ( Fig. 6 ). Colonic contents were gavaged into GF mice and their behaviour and microbiota profiles were assessed 3 weeks later. Illumina sequencing showed that the colonic microbiota composition was similar in mice gavaged with MS or control microbiota ( Fig. 6a ), which was in agreement with DGGE results showing a similarity index of 90–96% ( Supplementary Fig. 1d ). Similarly, we found no difference in the microbiota composition when analysing the OTUs relative abundance between colonized (gavaged) MS and control mice ( Supplementary Fig. 2c , summary at phylum level). Thus, the healthy mice that were gavaged with the gut microbiota of the dysbiotic mice ( Fig. 4 ) were not able to maintain that microbiota profile, which appears to shift towards normal in the healthy recipient mice. These results indicate that host factors present in MS mice, but absent in control mice, are required to select and maintain the microbiota associated with MS. The inability of healthy control mice to maintain the MS-associated microbiota was associated with a normal behavioural phenotype. Specifically, mice colonized with MS microbiota displayed behaviour similar to that of control mice in the step-down, light preference and tail suspension tests ( Fig. 6b–d ). As seen previously, bacterial colonization reduced the anxiolytic behaviour that characterizes GF mice when assessed by the light preference test ( Fig. 6d , F (1,13)=137.63, P <0.001). Similar results were observed when analysing only male mice ( Fig. 6b–d ). 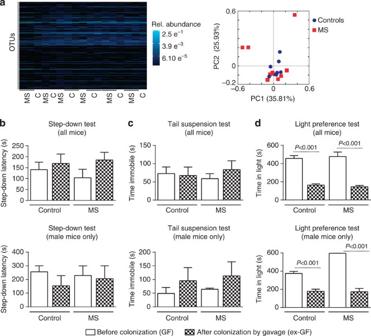Figure 6: Altered microbial and behaviour profiles were not transferred into control GF mice. (a) OTUs distribution at phylum level plotted in an ordination-organized heat map (based on Bray Curtis distance metric) of GF mice gavaged with faecal microbiota from MS or control mice (left panel). The data are normalized to proportional abundances and are represented by the intensity (blue) for each OTU. On the right, PCoA ordination plot of Morisita–Horn dissimilarity matrix calculated with QIIME on direct read counts of GF mice gavaged with faecal microbiota from MS or control mice (right panel). (b) Latency to step down from an elevated platform; (c) total duration of immobility during tail suspension test; (d) total time spent in the illuminated compartment during the light preference test in control healthy mice (upper panels), and male mice only (lower panels), before (GF) and after colonization (ex-GF) by gavage with control and MS microbiota. (MS,n=9, 5 males and 4 females; control,n=8, 2 males and 6 females). The graphs represent mean±s.e.m. The data were analysed with mixed two-way repeated measures ANOVA, where the between-subjects categorical variable was ‘microbiota’ (from MS or control SPF mice) and the within-subjects categorical variable was ‘colonization’ (before and after colonization). If a statistically significant effect of one of the categorical variables was observed, at-test within groups was performed. Rel. relative. Figure 6: Altered microbial and behaviour profiles were not transferred into control GF mice. ( a ) OTUs distribution at phylum level plotted in an ordination-organized heat map (based on Bray Curtis distance metric) of GF mice gavaged with faecal microbiota from MS or control mice (left panel). The data are normalized to proportional abundances and are represented by the intensity (blue) for each OTU. On the right, PCoA ordination plot of Morisita–Horn dissimilarity matrix calculated with QIIME on direct read counts of GF mice gavaged with faecal microbiota from MS or control mice (right panel). ( b ) Latency to step down from an elevated platform; ( c ) total duration of immobility during tail suspension test; ( d ) total time spent in the illuminated compartment during the light preference test in control healthy mice (upper panels), and male mice only (lower panels), before (GF) and after colonization (ex-GF) by gavage with control and MS microbiota. (MS, n =9, 5 males and 4 females; control, n =8, 2 males and 6 females). The graphs represent mean±s.e.m. The data were analysed with mixed two-way repeated measures ANOVA, where the between-subjects categorical variable was ‘microbiota’ (from MS or control SPF mice) and the within-subjects categorical variable was ‘colonization’ (before and after colonization). If a statistically significant effect of one of the categorical variables was observed, a t -test within groups was performed. Rel. relative. Full size image MS is a widely used model of early-life stress that results in the expression of anxiety- and depression-like behaviour in adulthood [4] , and our characterization of the behavioural phenotype of maternally separated mice is in keeping with published studies. However, our studies extend the findings of others showing alterations in the microbial composition in the gut [18] by demonstrating, for the first time, the critical contribution of the intestinal microbiota in the expression of the MS behavioural phenotype. We show that while changes in HPA axis activation and in colonic physiology are retained in GF MS mice, the anxiety- and depression-like behaviour is absent. However, the behavioural phenotype could be restored when microbiota from control (non-MS) mice was transferred into GF MS mice and modified by the colonic environment of MS mice. The importance of host factors, acting in conjunction with the microbiota, is further illustrated by our demonstration that the MS behavioural phenotype cannot be induced by simply colonizing control GF mice with the microbiota from MS mice. Thus, it is evident that the behavioural phenotype of this model of early-life stress reflects a convergence of microbial and host factors. While it is well established that MS produces long-lasting abnormalities in emotion-related behaviour in rodents with conventional microbiota, the abnormal behavioural profile depends on the species, strain, gender and experimental condition used [31] , [32] . Our earlier study demonstrated behavioural despair in MS mice using the tail suspension test [8] , [33] . In this study, using the step-down, light preference and tail suspension tests, we also show anxiety-like behaviour in SPF MS mice. These mice had increased aversion to the illuminated compartment and longer latency to re-enter this area, as well as a delayed latency to step down, features that are characterized as defensive or anxiety-like behaviours in rodents exposed to stressful events [34] , [35] , [36] . However, using three standard tests to assess anxiety-like behaviour and one test to evaluate behavioural despair [37] , GF MS mice displayed similar behaviour as GF controls, indicating that the gut microbiota is required for the development of anxiety-like behaviour and behavioural despair in the MS model. This was confirmed in the subsequent colonization experiments, which demonstrated a divergence of microbiota profiles and altered behaviour in ex-GF MS mice, but not in controls. Although prenatal stress related to the shipment of the pregnant SPF dams could contribute to the observed behavioural differences between GF and SPF mice, this would not apply to the ex-GF colonized mice, as they were raised and handled in our gnotobiotic facility. MS GF mice did not display anxiety-like behaviour, despite having higher serum corticosterone levels than controls, similar to SPF MS mice. It is known that MS rodents with conventional microbiota have a hyperactive HPA axis and altered corticosterone levels, corticotropin-releasing factor (CRF) mRNA expression in the paraventricular nucleus and glucocorticoid receptor density in the hippocampus [16] , [18] , [21] , [38] , [39] , [40] , [41] , [42] . Moreover, the CRF-receptor 1 has been reported to mediate acute and delayed stress-induced visceral hyperalgesia in maternally separated rats [43] , and systemic or central CRF administration is known to alter intestinal epithelial physiology [44] , colonic motility [45] and the composition of the intestinal microbiota [45] . Indeed, we observed elevated serum corticosterone levels in MS GF mice, confirming that MS also induces a long-lasting vulnerability to stress under GF conditions, meaning that a microbial stimulus is not needed to alter the HPA axis response. In agreement with previously published data, basal corticosterone levels were similar in GF and conventional mice [23] , but we cannot exclude the possibility that differences may have emerged had we measured corticosterone levels after a stressful challenge. GF MS mice exhibited higher levels of BDNF in the hippocampus, but not in the amygdala, compared with GF control mice, demonstrating that MS induces alterations in brain biochemistry, even under GF conditions. However, no differences in BDNF levels were found between SPF MS and control mice. Altered BDNF in the hippocampus and the amygdala has been previously associated with anxiolytic and antidepressant behaviour by us [26] and others [25] , [27] , but in the present study, we did not find a overall correlation between BDNF levels and mouse behaviour, except for the increased levels of hippocampal BDNF and decreased behavioural despair in MS GF male mice. Controversial results emerge from previous studies of hippocampal BDNF in SPF mice following MS: some reported higher [46] , [47] , [48] and others lower BDNF levels [9] , [49] , [50] in MS rodents. These controversies may thus represent a combined, and sometime opposing, effects of MS and gut microbiota on the brain and behaviour. We confirmed that GF mice (both control and MS) had higher levels of hippocampal serotonin, as recently reported by Clarke et al . [26] , and found that they had lower levels of hippocampal noradrenaline compared with SPF mice. This is in agreement with recent study showing that gut microbiota influences brain’s monoamine metabolism, and that GF mice have lower dopamine and noradrenaline turnover rates in the brainstem and striatum in comparison with ex-GF mice [51] . A confounding factor in our study, when comparing brain chemistry in GF and SPF mice, might be their different age. While GF mice were 9–10 weeks old, the SPF and the ex-GF (SPF colonized) mice were 16–20 weeks old. In a recent study, no differences were observed in behaviour and brain BDNF levels in SPF C57Bl/6 mice between 1–2 and 5–6 months of age [52] , which is in agreement with previous reports showing no detectable differences in brain chemistry between adult mice of this age group [53] . However, there is no comparable data on brain development and neurotransmitters levels in GF mice. The gut–brain axis enables bidirectional communication between the brain, the gut and the intestinal microbiota, and this signalling may involve not only neuroendocrine but also immunological mechanisms [22] . In this study, we observed no differences in the levels of immune cell infiltrate or inflammatory markers in the gut. In addition, body weight was similar between MS and control adult, suggesting that the changes in behaviour observed in MS SPF mice were not related to developmental alterations or sickness behaviour [54] . However, a marked increase in colonic acetylcholine release was observed in both GF and SPF MS mice compared with controls. This is in agreement with a previous study demonstrating a hypercholinergic state of the colon of MS rat pups [15] , which might also be implicated in the visceral hypersensitivity, dysmotility and altered colonic mucus secretion described previously in adult MS rats [12] , [13] , [29] , [55] . Interestingly, GF MS mice also displayed increased faecal pellet output during the open-field test. This measure has been previously reported as a parameter of stress-induced stimulation of the colon by sacral parasympathetic outflow [28] . Acetylcholine is the main excitatory neurotransmitter in the mammalian enteric nervous system and plays an important role in the control of digestive functions [56] , [57] , gut motility [58] and permeability [15] . Our data thus suggest that MS leads to increased activity of cholinergic nerves in the colon independently of the presence of bacteria. Interestingly, GF mice released less acetylcholine than SPF mice after KCl stimulation, and we speculate that altered enteric cholinergic function may contribute to the abnormal gut motility previously reported in GF animals [59] , [60] . SPF MS mice displayed marked colonic dysbiosis as previously shown by O'Mahony et al . [18] We propose that the dysbiosis seen in this model is multifactorial. First, it is possible that the disruption of dam-pup contact early in life, when the microbiota is being established, affects the microbiota composition. It is also plausible that increased cholinergic activity of enteric nerves alters colonic motility and secretion, changing the physico–chemical environment within the colon, which results in the selection of a modified microbiota. Based on our colonization experiments, the latter is the more likely possibility. Furthermore, it has been shown that altered HPA axis activity or stressor exposure can significantly affect gut microbial composition and activity [45] , [61] , [62] . The importance of host factors in the development and/or maintenance of the altered behaviour is underscored by the fact that the presence of an altered microbiota alone is insufficient to induce anxiety or behavioural despair in control ex-GF mice. In fact, GF MS mice presented a strikingly different environmental niche for microbiota than that of control GF mice, exhibiting altered basal HPA axis activity and altered colonic neural cholinergic activity, with likely altered gut motility, permeability, ion secretion, mucin production and even altered intestinal morphology [29] . Indeed, when GF MS and control mice were colonized with the same control SPF microbiota, MS mice selected a different microbiota profile compared with control mice and exhibited an altered behavioural profile. The precise mechanisms, by which gut bacteria affect behaviour, are unclear, but since no differences in immune system activation were observed between MS and control mice, they may occur through production of neuroactive metabolites. The inferred metabolomic profiles obtained from colonized MS and control mice revealed differences in the metabolism of the neurotransmitter glutamate and neurotransmitter precursor’s phenylalanine, tryptophan and tyrosine, as well as fatty acids. It has been shown that the short-chain fatty acids (SCFAs) not only affect brain activity but also lower the pH in the colon. This may influence the microbiota composition as some Clostridia ( Clostridium group XIVa) survive well in an acidic environment, whereas Bacteroidetes spp. experience progressive inhibition at reduced pH values [63] . The altered microbiota profile observed in our study could be also linked to altered proteolytic activity in the gut, which can subsequently affect the neural system [64] . Higher abundance of Coribacteriales has been previously associated with increased faecal protease activity [65] , while a decrease in Bacteroides has been linked to high faecal tryptic activity [66] . Although we have not identified the exact underlying mechanisms in this model, our results are in agreement with previous studies showing that bacteria can produce or alter the metabolism of neurotransmitters [51] , [67] , [68] , modify expression of multiple genes within the CNS [24] , [25] , modulate metabolism of tryptophan/kynurenine [26] , directly affect neural activity [69] and alter serum metabolomic profile [70] . Several studies published in the past 2 years have suggested that GF mice have less anxiety-like behaviour compared with SPF mice [24] , [25] , [27] . However, a very recent study reported that a short time exposure to the environment makes GF mice less anxious [51] . In our study, we observed that GF mice spent longer time than SPF mice in the illuminated compartment during the light/dark preference test, and shorter time immobile than SPF mice during the tail suspension test, indicating greater anxiolytic and anti-depressive behaviour as previously reported [24] , [25] , [26] , [27] . However, an opposite conclusion could be reached from the fact that our GF mice took longer to step down from the elevated platform than SPF mice during the step-down test. To further complicate the issue, there was no difference in behaviour of control mice before and after colonization when using the step down or the tail suspension tests. Thus, the discrepancies observed between studies may be owing to the type of behavioural test applied, the duration of bacterial colonization, different environmental conditions during testing between GF and conventional mice, and most importantly, owing to differences in the microbiota profile, as we know that specific bacteria can have either anxiogenic [71] or anxiolytic [69] , [72] effects. This highlights the importance of conducting experiments under well-controlled conditions, including paired comparisons before and after interventions. Our studies were performed in a strictly sterile environment within gnotobiotic isolators. This is particularly important in light of the ease with which GF mice can become contaminated when exposed to the environment during behavioural testing, as it is known that bacterial products rapidly induce changes in ENS function, which in turn could affect gut–brain signalling [69] . In summary, our study provides novel insights into the determinants of behavioural alterations induced by early-life trauma. Taking advantage of a widely used model of early-life stress we have shown that the gut microbiota is critical, but not sufficient, to induce the behavioural phenotype that characterizes MS model. Indeed, both microbial and host factors must converge to produce alterations in behaviour. The critical host factors are those that shape the habitat and therefore the composition of the intestinal microbiota. Animals GF C57BL/6N mouse breeding pairs were housed under axenic conditions in the Axenic Gnotobiotic Unit of McMaster University. SPF pregnant C57BL/6N mice were obtained from Taconic Farms (Hudson, NY, USA) on gestational days 15–16. GF breeding pairs and SPF dams were individually housed on a 12:12-h light–dark cycle with free access to food and water. All experiments were approved by the McMaster University Animal Care Committee. Behavioural testing of SPF or GF mice was conducted at 8 weeks of age, from 9:00 to 12:00 ( Fig. 7 ). For the colonization experiments, behavioural testing was conducted at 8 weeks of age in GF conditions, and 3 weeks after colonization in SPF conditions, from 9:00 to 12:00. Mice were then killed in the standardized manner from 9:00 to 11:00. 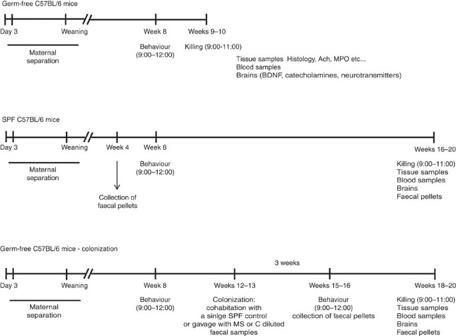Figure 7: Study design timeline. Schematic timeline representation of the GF, SPF and colonization experiments performed in the current study. Figure 7: Study design timeline. Schematic timeline representation of the GF, SPF and colonization experiments performed in the current study. Full size image Study design A timeline of the experiments is shown in Fig. 7 . SPF time-pregnant C57BL/6N female mice were obtained from Taconic Farms (Germantown, NY, USA) on gestational days 15–16. For GF experiments, the same strain of mice was re-derived in McMaster Axenic Gnotiobiotic Unit. The birth date was considered day 0. SPF and GF C57BL/6 mouse pups (entire litters) were randomly selected and exposed to MS as previously described [8] or left undisturbed in their cage (controls). Mouse behaviour was assessed at the same time of the day between 8 and 9 weeks of age. Mice were killed thereafter, with two control and two MS mouse killed daily, and intestinal content and tissue samples were collected. GF status of mice at the killing was verified by nucleic acid fluorescent stain (Sytox, Invitrogen, Burlington, ON), PCR and culture techniques. Male mice were used in SPF conditions [8] to prevent biological variations during behavioural tests. However, owing to limited GF mouse availability, both males and females were used and a possible gender effect was evaluated. MS pups were separated from the dam for 3 h per day (from postnatal day 4 until weaning), and placed into a new cage, whereas control pups remained in their home cage with the dam. The dams of the MS mice were transferred to separate holding cages during the MS procedure. The MS procedure in GF mice was identical except that it was carried out in gnotobiotic isolators under strict axenic conditions. For behavioural experiments in GF conditions, we used overall 54 control mice (15 litters) and 37 MS (8 litters) mice obtained over 3-year period (2011–2013). For behavioural experiments in SPF conditions, we used 20 SPF male control (5 litters) and 13 SPF male MS mice (7 litters), obtained over 1-year period (2008). For acetylcholine release experiments and corticosterone determinations, we used 16 GF control (4 litters), 13 GF MS (3 litters) (obtained between June 2011 and February 2012), and 20 SPF control (5 litters) and 13 SPF MS mice (7 litters) (obtained in 2008). Litter size in GF conditions is not as stable and predictable as in SPF conditions, and it ranges between 1 and 6 pups. At 12–13 weeks of age, two litters from each GF group, MS ( n =11) and control ( n =16), were colonized with normal SPF microbiota. The mice caged separately by gender and treatment were co-housed for a brief period of time (15 min) with two control SPF C57BL/6 female (11 weeks old) mice. The dirty bedding, water and food from the SPF female cage were divided between the GF cages to facilitate the colonization. Thereafter, the mice were maintained in gnotobiotic conditions for 3 weeks, until the behaviour testing. At 12–13 weeks of age, three extra GF litters ( n =17) were gavaged with SPF microbiota either from a control or a MS mouse. The mice caged separately by gender and treatment and maintained in gnotobiotic conditions for 3 weeks, until the behaviour testing. Behaviour assessment Anxiety-like behaviour was assessed using a light/dark preference test as previously described [54] using an automated system (Med Associates, St Albans, Vermont) or a custom-built apparatus equipped with a digital video camera. Both systems (arenas) had similar dimensions, and the behaviour was analysed in the identical fashion. Briefly, each mouse was placed in the centre of an illuminated box connected to a smaller dark box, and its behaviour was recorded for 10 min. Total time spent in the illuminated area, latency to re-enter light area, total distance travelled and average velocity were assessed. The step-down test was performed as described previously [36] . Briefly, each mouse was placed in the centre of an elevated platform, and latency to step down from the pedestal was measured (maximum 5 min). Behaviour assessment of GF mice was performed under strict axenic conditions using an automated system (Med Associates) customized to fit within the gnotobiotic isolator. Axenic mice of any strain are re-derived by embryo transfer technique at the large Axenic Gnotobiotic Unit at McMaster University. Experimental mice for behaviour assessment are housed in a dedicated sterile isolator within the Unit. Behavioural equipment, such as step-down platform, tail suspension device and light preference test inserts ( Supplementary Fig.8 ) are sterilized by autoclaving and then imported into a custom-made sterile isolator following the strict standard operating procedures of our Unit. For the light preference test, mouse behaviour in the apparatus inside the isolator is monitored by infrared beams and transmitted directly to a computer outside the isolator ( Supplementary Fig. 8 ). After each import of autoclaved material, sentinel mice in the isolator are tested using culture, fluorescence and molecular techniques. In addition to step-down and light preference tests, the mice also underwent the open-field and the tail suspension tests. In the open-field test, each mouse was placed in the centre of an open arena (29.2 × 29.2 cm) and behaviour was recorded for 10 min using an automated system (Med Associates). Total time spent in the centre (16% of the total area) and sides, and locomotor activity were assessed. Faecal pellet counts at the end of each test were used as a measure of the autonomic regulation of colonic motility [28] , [73] . During the tail suspension test, a measure of behaviour despair [37] , mice were suspended by their tails 30 cm above the ground from the custom-built device, and total duration of immobility (absence of body movement, hanging passively) was recorded during 5 min. This test is considered a ‘dry’ version of the forced swim test and it has been widely used to measure antidepressant drugs effectiveness [37] . Behavioural testing in SPF or GF conditions was conducted on 8-week-old mice always from 9:00 to 12:00. For the colonization experiments, behavioural testing was conducted at 8 weeks of age in GF conditions, and 3 weeks after colonization in SPF conditions, always from 9:00 to 12:00. Longitudinal muscle–myenteric plexus preparation assay The colon was removed and cut in half. Longitudinal muscle–myenteric plexus preparations were dissected, placed in oxygenated Krebs’ solution and pre-incubated with 0.5 μmol l −1 of [3H]-choline for 40 min at 37 °C as previously described [74] . Tissues were then transferred to superfusion chambers and perfused with Krebs’ solution with 5 mM hemicholinium-3 (ref. 75 ) at a rate of 1 ml min −1 . Aliquots were collected every 2 min for 80 min using Altrorac 7000 fraction collector (LKB, Stockholm, Sweden). [3H]-Acetylcholine release was induced by EFS (30 V, 10 Hz, 0.5 mS) for 1 min (S48 stimulator; Grass, Quincy, MA) or by adding 50 mmol/l KCl to the superfusate for 6 min, and then measured using a Beckman scintillation counter (LS5801; Beckman Instruments, Fullerton, CA) at a counting efficiency of 35% and expressed as a fraction of the total [3H] in the tissue. Histology Colonic tissue samples fixed in 10% buffered formalin were embedded in paraffin. Tissue sections were stained with haematoxylin and eosin, and inflammation was evaluated by a blinded observer. Assessment of inflammation and corticosterone Blood was collected under isoflurane (Abbott Laboratories, Saint-Laurent, Québec, Canada) anaesthesia by cardiac puncture; serum was separated and stored at −80 °C. C-reactive protein was measured with ELISA kit (ICL, Newberg, OR, USA) and corticosterone with RIA kit (MP Biomedicals, Santa Ana, CA, USA). Additional samples were snap-frozen in liquid nitrogen for assessment of MPO activity. MPO assay was performed as described previously [69] and its activity was expressed in units per milligrams. BDNF and catecholamine analysis Brains were collected and frozen in cooled 2-methylbutane (Sigma, Canada) and stored at -80 °C. BDNF analysis on the hippocampus and the amygdala regions was performed as previously described [27] . BDNF was measured using two-site ELISA (BDNF Emax immunoassay system; Promega, Madison, WI). The protein concentration was measured by BCA protein assay kit (Bio-Rad, Mississauga, ON, Canada). Results were expressed as pg of BDNF per mg of protein. For catecholamine and serotonin analysis, the amygdala and the hippocampus were isolated as previously described for BDNF analysis [27] . The sections were diluted 1:10 (weight:volume) with 0.01 N HCl in the presence of EDTA (1 mM) and sodium metabisulfite (4 mM; Sigma) at a pH >7. For serotonin evaluation, 1% stabilizer was added to the buffer according to manufacturer’s instructions. Noradrenaline, dopamine and serotonin were then measured in the sections with the 2-cat Research ELISA kit and Serotonin Research ELISA kit (LDN, Nordhorn, DE). DGGE analysis Faecal samples were collected at 4 and 20 weeks of age from SPF control and MS mice for further analysis of the gut microbiota composition (DGGE analysis and Illumina). Similarly, faecal pellets were collected from colonized ex-GF control and MS mice 3 weeks after colonization for further analysis of the gut microbiota composition (DGGE analysis and Illumina). The V2–V3 region of the 16S ribosomal DNA gene of bacteria in the colonic content of ex-GF control and MS mice was amplified with primers HDA1-GC and HDA2 (ref. 76 ) and performed as previously reported [27] . Gel Compar II software (Applied Maths, Austin, TX, USA) and Quantity One software (version 4-2; Bio-Rad Laboratories) were used to analyse the DGGE gels. DGGE analysis allows for α- and β-diversity analysis (within- and between-community diversity, respectively). The relatedness of microbial communities was expressed as similarity clusters, using the Dice coefficient and the unweighted- and weighted-pair (UPGMA and WPGMA) group method using average linkages. Deep-sequencing analysis of 16S rRNA with Illumina The V3 region of the 16S rRNA gene was amplified as previously described [77] , [78] . Briefly, 100 mg of faecal or caecal sample were resuspended in 1 ml of a solution of PBS and guanidine thiocyanate–ethylenediaminetetraacetic acid–Sarkosyl (9:1), and homogenized using 0.2 g of 0.1-mm glass beads (Mo Bio, Carlsbad, CA). Enzymatic lysis and a phenol–chloroform–isoamyl alcohol extraction were performed followed by a clean-up step (Zymo, Irvine, CA). After separating the products from primers and primer dimers by electrophoresis on a 2% agarose gel, PCR products of the correct size were recovered using a QIAquick gel extraction kit (Qiagen, Mississauga, ON, Canada). A total of 16,639,036 reads before quality filtering (an average of 386,954 reads per sample with a range of 7,514–1,014,894), 6,766,046 reads after quality filtering (an average of 157,350 reads per sample with a range of 2,757–417,514) and 1,184 OTUs (an average of 211.83 OTUs per sample with a range of 38–449 OTUs per sample, after quality filtering) were obtained from the 43 samples sequenced (Bioproject PRJNA264561, SRA accession code SRP049244 ). The samples included were as follows: 8 samples from SPF mice (4 controls and 4 MS), 17 samples from mice colonized by gavage (8 controls and 9 MS), 18 samples from mice colonized through cohabitation (donor 1: 3 controls and 4 MS; donor 2: 4 controls and 7 MS). Custom, in-house Perl scripts were developed to process the sequences after Illumina sequencing [78] . Cutadapt [79] was used to trim any over-read, and paired-end sequences were aligned with PANDAseq [80] with a 0.7 quality threshold. If a mismatch in the assembly of a specific set of paired-end sequences was discovered, they were culled. In addition, any sequences with ambiguous base calls were also discarded. OTUs were picked using AbundantOTU+ [81] , and sequences were clustered to 97% sequence identity OTUs. Taxonomy was assigned at a 0.8 threshold using the Ribosomal Database Project [82] classifier v.2.2 trained against the Greengenes SSU database (February 2011 release). For all downstream analyses, we filtered the obtained OTU table excluding ‘Root’ and excluding any sequence that was not present at least three times across the entire data set. Calculations of within-community diversity (α-diversity) and between-community diversity (β-diversity) were run using QIIME [82] , and the phyloseq package (version 1.8.2) implemented in R (version 3.1.0; ref. 83 . The graphics in Figs 2a , 4a,b and 6a (left panels) were produced using the phyloseq package (version 1.8.2) implemented in R (version 3.1.0), with the ‘plot_heatmap()’ function. The ordination method used in the plot_heatmap() function was the PCoA, and the metric used was Bray Curtis. For this function, the data were converted to relative data with the following script: Reldata=transform_sample_counts(phyloseqdata, function(x) x/sum(x)). The graphics in Figs 2a , 4a,b and 6a (right panels) were produced ordinating the dissimilarity matrix previously calculated with the Morisita–Horn method in a PCoA plot using QIIME, which uses direct read counts and accounts for different sample depth. For the statistical analyses on the taxonomic composition, first we used the script otu_category_significance.py in QIIME, which determines using ANOVA whether OTU relative abundance is different between categories. This script automatically removes OTUs that are not found in at least 25 per cent of samples and corrects the P values obtained from the comparison between categories (controls versus MS) with the ‘false discovery rate’ (FDR) method. Second, we analysed the taxonomic composition of the samples with multiple t -tests on the table L6 (the highest assigned taxonomic level) generated by running the script: summarize_taxa_through_plots.py in QIIME. The P values obtained from the comparison between groups (controls versus MS) were corrected with the ‘FDR’ method, accepting a 3% FDR. All the samples were run twice and analysed twice to confirm the results obtained. The prediction of the functional composition of a metagenome using marker gene data and a database of reference genomes was done with PICRUSt as described by Langille et al . [30] . The graphical representation of the results was done with STAMP [84] and the calculation of P values was done with White’s non-parametric t -test, applying Storey FDR correction [85] . Statistical analysis Statistical analysis was performed using SPSS 20.0 software for Windows (SPSS Inc., Chicago, IL, USA). The data for all mice (pooled males and females) and males only are presented separately to minimize the gender effect and shown as mean±s.e.m. or medians (Interquartile Deviation Method). Statistical comparisons were performed using ANOVA, Mann–Whitney test or multiple t -test, as appropriate. Two-way repeated measures ANOVA was used to compare GF and colonized mice, whereas a two-way ANOVA was used to compare GF and SPF mice. When using two-way ANOVA, a statistical significant effect of a factor was found, then differences within groups were analysed with t -test. Benjamini and Hochberg FDR correction method was used when multiple comparisons were performed. P value of <0.05 was considered statistically significant. Detailed description of the statistical methods was included in the pertinent result section. Accession codes: The microbiome sequence data have been deposited in the Bioproject and the Sequence Read Archive databases with accession codes PRJNA264561 and SRP049244 , respectively. How to cite this article: De Palma, G. et al . Microbiota and host determinants of behavioural phenotype in maternally separated mice. Nat. Commun. 6:7735 doi: 10.1038/ncomms8735 (2015).